Unexpected reactivity and mechanism of carboxamide activation in bacterial N-linked protein glycosylation The initial glycan transfer in asparagine-linked protein glycosylation is catalysed by the integral membrane enzyme oligosaccharyltransferase (OST). Here we study the mechanism of the bacterial PglB protein, a single-subunit OST, using chemically synthesized acceptor peptide analogues. We find that PglB can glycosylate not only asparagine but also glutamine, homoserine and the hydroxamate Asp(NHOH), although at much lower rates. In contrast, N -methylated asparagine or 2,4-diaminobutanoic acid (Dab) are not glycosylated. We find that of the various peptide analogues, only asparagine- or Dab-containing peptides bind tightly to PglB. Glycopeptide products are unable to bind, providing the driving force of product release. We find no suitably positioned residues near the active site of PglB that can activate the acceptor asparagine by deprotonation, making a general base mechanism unlikely and leaving carboxamide twisting as the most likely mechanistic proposal for asparagine activation. The biosynthesis of N-linked glycoproteins is a fundamental post-translational process in eukaryotes. It occurs at the membrane of the endoplasmic reticulum, where the multimeric integral membrane enzyme oligosaccharyltransferase (OST) catalyses the covalent attachment of an oligosaccharide to asparagine residues of nascent polypeptide chains. As N-linked glycosylation is essential for a multitude of cellular processes, deletion of OST in eukaryotes is lethal [1] , [2] , [3] , [4] , [5] . Protein N-glycosylation is common in Archaea [6] , [7] , [8] and has also been found in defined taxa of Bacteria [9] , [10] , [11] . In prokaryotes, OST is a single subunit enzyme that is homologous to the catalytic STT3 subunit of eukaryotic OST. The glycan donor of the transfer reaction is a lipid-linked oligosaccharide (LLO), whereas the acceptor is an asparagine residue located in the consensus sequon Asn-Xaa-Ser/Thr (with Xaa≠Pro) [12] . Given the high degree of sequence similarity, the key steps of the reaction mechanism of N-linked glycosylation are probably conserved. This includes the catalytic activation of the generally unreactive amide group of the acceptor Asn to serve as a nucleophile attacking the C1 carbon of the LLO molecule, resulting in a nucleophilic substitution ( Fig. 1 ). 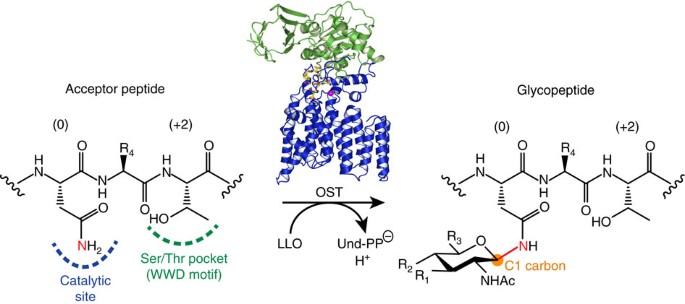Figure 1: The reaction catalysed by oligosaccharyltransferase. An acceptor polypeptide containing the consensus sequence Asn-Xaa-Ser/Thr is recognized by OST and the side chain amide of the asparagine is activated for a nucleophilic attack on a LLO (α-linkage). The inversion reaction results in the formation of a β1–N-glycosidic linkage (red bond) between the asparagine side chain and the C1 carbon of the reducing end sugar (orange circle), as well as the release of lipid pyrophosphate and one proton. Asn and Thr are indicated as (0) and (+2) sequon position, respectively. The bacterial OST fromC. lariis shown as ribbon diagram (PDB code 3RCE) with the transmembrane domain coloured in blue, periplasmic domain in green, acceptor peptide in yellow and divalent metal cation as a purple sphere. R1: OH (eukaryotes), Oligosaccharyl (bacteria); R2: Oligosaccharyl (eukaryotes), NHAc (bacteria); R3: CH2OH (eukaryotes), CH3(bacteria); R4: Xaa (≠Pro). Figure 1: The reaction catalysed by oligosaccharyltransferase. An acceptor polypeptide containing the consensus sequence Asn-Xaa-Ser/Thr is recognized by OST and the side chain amide of the asparagine is activated for a nucleophilic attack on a LLO (α-linkage). The inversion reaction results in the formation of a β1–N-glycosidic linkage (red bond) between the asparagine side chain and the C1 carbon of the reducing end sugar (orange circle), as well as the release of lipid pyrophosphate and one proton. Asn and Thr are indicated as (0) and (+2) sequon position, respectively. The bacterial OST from C. lari is shown as ribbon diagram (PDB code 3RCE) with the transmembrane domain coloured in blue, periplasmic domain in green, acceptor peptide in yellow and divalent metal cation as a purple sphere. R 1 : OH (eukaryotes), Oligosaccharyl (bacteria); R 2 : Oligosaccharyl (eukaryotes), NHAc (bacteria); R 3 : CH 2 OH (eukaryotes), CH 3 (bacteria); R 4 : Xaa (≠Pro). Full size image To explain this unusual reactivity, a direct involvement of the +2 Ser/Thr of the sequon was previously proposed [12] , [13] , [14] . This was notably inconsistent with the X-ray structure of a complete bacterial OST, the PglB protein from Campylobacter lari , which showed that the acceptor Asn and the +2 Ser/Thr are physically separated and that the +2 Thr is tightly bound to the WWD motif, a conserved and diagnostic motif in STT3 proteins [15] , [16] . This excluded an involvement of the hydroxyl amino acid in acceptor asparagine activation. Given the location of the catalytically essential divalent metal ion and the conserved carboxyl groups of Asp56 and Glu319 in the PglB structure, we proposed that a rotation of the C-N bond twisted the carboxamide group of the acceptor Asn, which would abolish the conjugation of the nitrogen lone pair with the carbonyl group, resulting in a highly reactive nucleophile [16] . To probe the mechanistic hypotheses, we perform in vitro analyses of C. lari PglB. We synthesize a series of fluorescently labelled peptides with various non-natural amino acids replacing the acceptor Asn and purify large quantities of wild-type and mutant PglB. We take advantage of a previously established assay that not only provides high precision in determining glycosylation turnover but also allows us to observe very low reaction rates of disfavoured PglB mutants [15] . We also quantify the first step of the in vitro glycosylation reaction, peptide binding, using fluorescence anisotropy. We find that PglB is able to perform unexpected reactions, as it also catalyses the formation of O-glycosidic linkages. Our studies provide biochemical evidence that is inconsistent with every postulated reaction mechanism except the ‘twisted amide’ activation of the acceptor asparagine. We therefore conclude that carboxamide twisting is most likely a key step during protein N-glycosylation. The amide group of Asn contributes to substrate binding The PglB structure revealed specific contacts between bound substrate peptide and the surface of the enzyme, including interactions involving the −2 and +2 sequon positions, but also between the acceptor Asn and the catalytically important PglB residues Asp56 and Glu319 [16] . We recently showed that mutations D56A and E319A not only reduced the catalytic activity but also impaired substrate peptide binding significantly [15] . We now replaced Asn in the glycosylation sequon DQ N AT of substrate peptides by structurally modified analogues and quantified the effect on peptide binding and glycosylation turnover. We observed that replacing Asn by Ala strongly reduced peptide binding, with K d too low to be determined in our assay ( Table 1 compound 2, Fig. 2a ). We conclude that, whereas the side chain of Ala can be accommodated in the tunnel connecting the peptide-binding and the catalytic sites of PglB, there are strong interactions to the enzyme that were removed along with the carboxamide group. When the acceptor Asn was replaced by Asp, peptide binding was still impaired ( Table 1 , compound 3, Fig. 2a ), suggesting that the negative charge of the carboxyl group causes electrostatic repulsion with residues Asp56 and Glu319. Our in vitro glycosylation assay also showed no glycopeptide formation of compound 3, confirming previous reports that Asp is no glycosylation acceptor for eukaryotic OST (ref. 17 ). Table 1 Turnover rates and peptide binding for acceptor asparagine analogues. 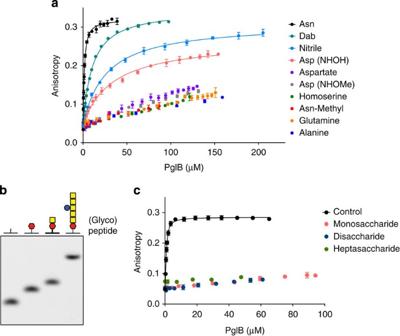Figure 2: Peptide binding of different acceptor asparagine analogues and glycopeptides. (a) Peptide binding was quantified using fluorescence anisotropy. Purified PglB was titrated into a solution containing 1 μM fluorescently labelled peptide variant (containing the sequon DQXAT with X=Asn or Asn analogue as indicated in the figure) and 10 mM MnCl2. Data points reflect the mean of 20 measurements of the same sample, error bars indicate s.d.’s. Data for Asn peptide (black curve) are as presented in Gerberet al.15(b) SDS–PAGE analysis ofin vitroglycosylation using fluorescently labelled substrate peptide (DQNAT sequon) and LLOs with different glycan structures. Depending on the presence and size of the N-glycan, peptides show a different mobility after Tricine SDS–PAGE. Bands were visualized using a fluorescence gel scan (488 nm excitation and 526 nm emission). Red hexagon: di-N-Acetyl-bacillosamine (diNAcBac); yellow square:N-Acetyl-galactosamine (GalNAc); blue circle: glucose. (c) Quantification of peptide and glycopeptide binding using fluorescence anisotropy. Samples were extracted fromin vitroglycosylation reactions. Treatment and data processing as in (a). Curve fitting for non-glycosylated peptide (control) was performed assuming a single binding site (R2=0.995). Full size table Figure 2: Peptide binding of different acceptor asparagine analogues and glycopeptides. ( a ) Peptide binding was quantified using fluorescence anisotropy. Purified PglB was titrated into a solution containing 1 μM fluorescently labelled peptide variant (containing the sequon DQ X AT with X=Asn or Asn analogue as indicated in the figure) and 10 mM MnCl 2 . Data points reflect the mean of 20 measurements of the same sample, error bars indicate s.d.’s. Data for Asn peptide (black curve) are as presented in Gerber et al . [15] ( b ) SDS–PAGE analysis of in vitro glycosylation using fluorescently labelled substrate peptide (DQ N AT sequon) and LLOs with different glycan structures. Depending on the presence and size of the N-glycan, peptides show a different mobility after Tricine SDS–PAGE. Bands were visualized using a fluorescence gel scan (488 nm excitation and 526 nm emission). Red hexagon: di- N -Acetyl-bacillosamine (diNAcBac); yellow square: N -Acetyl-galactosamine (GalNAc); blue circle: glucose. ( c ) Quantification of peptide and glycopeptide binding using fluorescence anisotropy. Samples were extracted from in vitro glycosylation reactions. Treatment and data processing as in ( a ). Curve fitting for non-glycosylated peptide (control) was performed assuming a single binding site ( R 2 =0.995). Full size image PglB processes glutamine residues A Gln in the ‘zero position’ of a glycosylation sequon should in principle provide a carboxamide group. However, Gln residues are generally not glycosylated. The PglB structure suggested that compared with Asn, the side chain of Gln would reach beyond the catalytic pocket. Alternatively, with the carboxamide group of Gln properly aligned in the active site, contacts between the acceptor peptide backbone and PglB would have to be abolished. We indeed found that binding of the Gln-containing peptide (compound 4) was as weak as that of the alanine-containing peptide ( Table 1 , compound 4, Fig. 2a ). Nevertheless, compound 4 could be glycosylated, albeit at a rate that was ~200,000-fold reduced compared with the Asn-containing sequon ( Table 1 , compound 4). To ensure that the generated glycopeptide was indeed the postulated ‘Q-linked’ product, we elevated the enzyme concentration such that the conversion of the Gln-peptide was about 40% complete ( Fig. 3a ), thus generating sufficient product for the MS analysis. MS spectra of the extracted glycopeptide were consistent with the C. jejuni N-glycan attached to the Gln-containing sequon ( Fig. 3b–d ). A subsequent MS3 sequencing analysis demonstrated that the glycan was attached to the second (underlined) Gln of the acceptor sequon DQ Q AT, fulfilling substrate specificities at the −2 and +2 positions of the sequon ( Supplementary Fig. S1 ). These findings demonstrate that the carboxamide group of an OST substrate has to be properly positioned in the active site for binding and activation. 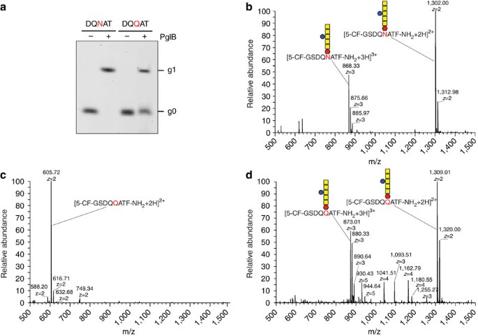Figure 3: Glutamine glycosylation catalysed by PglBin vitro. (a) Analysis ofin vitroglycosylation using fluorescently labelled substrate peptide containing either a DQNAT or a DQQAT acceptor site. Glycosylated peptide (g1) is separated from non-glycosylated peptide (g0) after Tricine SDS–PAGE. Bands were visualized using a fluorescence gel scan (488 nm excitation and 526 nm emission). (b) LC-ESI-MS profile of extracted glycopeptide (reaction with PglB) containing the DQNAT site. The doubly charged (m/z=1,302.0) and triply charged (m/z=868.33) glycopeptides are indicated. (c) LC-ESI-MS profile of doubly charged peptide (m/z=605.72) (reaction w/o PglB) containing the DQQAT site. (d) LC-ESI-MS profile of extracted glycopeptide (reaction with PglB) containing the DQQAT site. The doubly charged (m/z=1,309.01) and triply charged (m/z=873.01) glycopeptides are indicated. (b–d) Red hexagon: diNAcBac; yellow squares: GalNAc; blue circles: glucose; 5-CF: 5-carboxyfluorescein. Figure 3: Glutamine glycosylation catalysed by PglB in vitro . ( a ) Analysis of in vitro glycosylation using fluorescently labelled substrate peptide containing either a DQ N AT or a DQ Q AT acceptor site. Glycosylated peptide (g1) is separated from non-glycosylated peptide (g0) after Tricine SDS–PAGE. Bands were visualized using a fluorescence gel scan (488 nm excitation and 526 nm emission). ( b ) LC-ESI-MS profile of extracted glycopeptide (reaction with PglB) containing the DQ N AT site. The doubly charged (m/z=1,302.0) and triply charged (m/z=868.33) glycopeptides are indicated. ( c ) LC-ESI-MS profile of doubly charged peptide (m/z=605.72) (reaction w/o PglB) containing the DQ Q AT site. ( d ) LC-ESI-MS profile of extracted glycopeptide (reaction with PglB) containing the DQ Q AT site. The doubly charged (m/z=1,309.01) and triply charged (m/z=873.01) glycopeptides are indicated. ( b – d ) Red hexagon: diNAcBac; yellow squares: GalNAc; blue circles: glucose; 5-CF: 5-carboxyfluorescein. Full size image PglB catalyses the formation of O-glycosidic linkages We hypothesized that oxygen atoms could serve as nucleophiles as long as they are not negatively charged. We thus replaced Asn with homoserine (Hse) in the acceptor sequon (compound 5). Even though the hydroxyl group of Hse could in principle form one hydrogen bond to the active site residue Asp56 or Glu319, peptide binding was as weak as for the Ala-containing peptide ( Table 1 , compound 5, Fig. 2a ). However, we found that compound 5 was glycosylated by PglB, with a turnover rate ~900-fold slower than wild-type (wt) sequon. PglB can thus generate an O-glycosidic linkage if the corresponding acceptor site is positioned correctly for a nucleophilic attack on the LLO donor. We also analysed peptides with substituents attached to the carboxamide group of the acceptor Asn. Replacing one amide proton by a hydroxyl group (yielding the hydroxamate Asp(NHOH), compound 6) led to a reduced binding affinity ( K d of 33±2.4 μM), whereas an analogous replacement with a methyl group (Asn-Me, compound 7) or an O-methyl group (Asp(NHOMe), compound 8) prevented peptide binding altogether ( Table 1 , Fig. 2a ). Compounds 7 and 8 did not serve as substrates for PglB. In contrast, the hydroxamate compound 6 was glycosylated ~20 times slower than wt sequon ( Table 1 ). An analysis of the glycosylated compound 6 using matrix-assisted laser desorption/ionization-mass spectrometry (MALDI-MS) yielded a mass consistent with the C. jejuni N-glycan attached to the Asp(NHOH) peptide ( Supplementary Fig. S2 ). To identify the glycan attachment point, we analysed the resulting glycopeptide using NMR spectroscopy. The assignment of 13 C– 1 H heteronuclear single-quantum correlation (HSQC) spectra confirmed the presence of all expected signals for compound 6 in the educt and product ( Supplementary Fig. S3 ). The attached bacterial glycan shows signals similar to those observed for in vitro glycosylated AcrA protein [18] , except for the C1–H1 correlation of di- N -Acetyl-bacillosamine (diNAcBac) ( Supplementary Fig. S4 ). The characteristic chemical shift of C1 involved in the N-glycan linkage of ~81 p.p.m. was missing [18] , [19] , [20] . Instead, the C1 chemical shift of diNAcBac was assigned to 106.4 p.p.m. by first identifying the associated H1 chemical shift using two-dimensional (2D) nuclear Overhauser enhancement spectroscopy (NOESY) and 2D total correlation spectroscopy (TOCSY) spectra and subsequently a C1–H1 correlation in a 1 H- 13 C-HSQC spectrum ( Supplementary Figs S4, S5 ). This unusual chemical shift for the anomeric C1 of diNAcBac is incompatible with an N-glycan and rather suggests an O-glycosidic linkage. Almost identical C1 values were indeed reported for O-linked glycosyl hydroxamates [21] , [22] . Thus, the oxygen atom of the hydroxamate compound Asp(NHOH) was glycosylated by PglB, resulting in an O-glycosidic bond. Owing to the alpha effect, compound 6 (hydroxamate) is a better nucleophile than the Hse-containing compound 5 (ref. 23 ), even though the positioning of the hydroxyl group of Asp(NHOH) in the active site is not optimal (similar to glutamine). Inhibitor peptides and product glycopeptides Replacing the acceptor Asn in the sequon by the corresponding primary amine results in the residue 2,4-diaminobutanoic acid (Dab), which was reported to have inhibitory effects on eukaryotic OST [14] , [24] . We determined a K d of 10±0.25 μM for a synthetic peptide containing Dab at the acceptor position ( Table 1 , compound 9, Fig. 2a ), which is ~10-fold weaker binding than wt sequon. However, we observed no glycosylation of compound 9, even at elevated enzyme concentrations. Replacing the carboxamide group of Asn by a nitrile group also abolished glycosylation, although the peptide analogue bound with a K d of 26±1.6 μM ( Table 1 , compound 10, Fig. 2a ). Consequently, peptides containing the Dab or the nitrile group at the acceptor position of sequons represent competitive inhibitors for PglB. We further investigated whether N-linked glycopeptides reflecting the products of PglB-catalysed glycosylation could still bind the enzyme. To study distinct glycan structures, we took advantage of engineered versions of the C. jejuni pgl gene cluster, which yielded LLO donors containing a trisaccharide (GalNAc-α-1,4-GalNAc-α1,3-diNAcBac-α1-PP-Und) or a disaccharide (GalNAc-α1,3-diNAcBac-α1-PP-Und) [25] . We used extracts of these LLO variants along with wt C. jejuni LLO to glycosylate compound 1 in vitro . The trisaccharide was subsequently trimmed by an established glycosidase treatment [26] to yield a monosaccharide-containing LLO molecule ( Supplementary Fig. S6 ). Non-glycosylated peptide and peptides containing mono-, di- and heptasaccharide covalently attached to the acceptor asparagine were extracted from the reaction mixture ( Fig. 2b ). Fluorescence anisotropy analysis revealed that only the unmodified peptide bound to PglB ( Fig. 2c ), supporting the notion that the presence of a β1-linked N-glycan may cause steric tension in the catalytic site, triggering product release [16] . This is distinct to the findings with O-GlcNAc transferase, which can bind product glycopeptides [27] , [28] . Active site mutations The previously suggested mechanisms of Asn activation postulated an essential catalytic base [12] , [13] , [14] . In PglB, the side chain of His485 provides the only potential base located in the expected direction of the nucleophilic attack ( Fig. 4a ). His485 is only conserved in bacterial PglB proteins. The equivalent residue in archaeal OST is a glutamine, and eukaryotic STT3 proteins feature a tryptophan ( Supplementary Fig. S7 ). Compared with the wt PglB, we found only slightly reduced activities of the mutants H485A, H485L and H485F in an in vivo glycosylation assay, and activities reduced to ~30% in the mutants H485D and H485Q ( Fig. 4b ). These findings exclude a role of His485 as an essential catalytic base. The absence of activity of mutant H485W ( Fig. 4b ) is attributed to steric hindrance, with the large tryptophan side chain disturbing the structure or acceptor Asn binding ( Fig. 4a ). Our efforts to determine sequon affinities to His485 mutants failed because the studied mutants proved unstable in detergent solution, suggesting that His485 has a structural rather than a functional role, possibly by stacking against Trp464, which is part of the WWD motif ( Fig. 4a ). 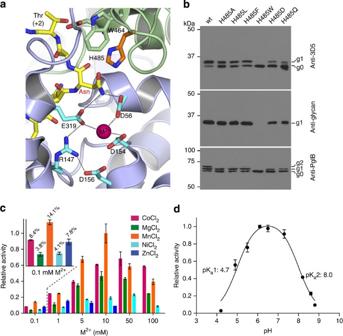Figure 4: PglB catalytic site studies. (a) Structure of PglB-active site (PDB code 3RCE). Transmembrane and periplasmic domains are coloured in light blue and green, respectively. Selected side chains are labelled and are shown in ball and stick with transmembrane domain residues coloured in cyan, periplasmic domain residues coloured in green or orange (H485) and acceptor peptide coloured in yellow. Grey dashed lines indicate putative hydrogen bonds or interactions with the divalent metal cation M2+(purple sphere). (b)In vivoglycosylation assay inE. colito investigate the functional importance of residue His485. Immunoblots detecting acceptor protein 3D5 (top), bacterial N-glycans (middle) and PglB (bottom). PglB mutants are indicated above the lanes. Glycosylation results in a mobility shift from the non-glycosylated (g0) to the glycosylated form of the acceptor protein (g1). Functional PglB is partially auto-glycosylated at N535 and N556, resulting in two additional bands (g1 and g2). (c) Influence of different divalent metal cations onin vitroactivity of PglB. The turnover rate of PglB devoid of the His10affinity tag on fluorescently labelled substrate peptide (DQNAT sequon) was determined at various concentrations of different divalent metal cations. The activity profile at 0.1 mM metal concentration is magnified in the inlet. (d) pH activity profile of PglB. The turnover rate of PglB on fluorescently labelled substrate peptide (DQNAT sequon) was determined at various pH values and the obtained data were fitted with a function describing a bell-shaped pH curve (R2=0.976). The calculated pKavalues are indicated. (c,d) Each data point results from a single turnover rate determination and the error bars account for the s.e.m. of each fit. Figure 4: PglB catalytic site studies. ( a ) Structure of PglB-active site (PDB code 3RCE). Transmembrane and periplasmic domains are coloured in light blue and green, respectively. Selected side chains are labelled and are shown in ball and stick with transmembrane domain residues coloured in cyan, periplasmic domain residues coloured in green or orange (H485) and acceptor peptide coloured in yellow. Grey dashed lines indicate putative hydrogen bonds or interactions with the divalent metal cation M 2+ (purple sphere). ( b ) In vivo glycosylation assay in E. coli to investigate the functional importance of residue His485. Immunoblots detecting acceptor protein 3D5 (top), bacterial N-glycans (middle) and PglB (bottom). PglB mutants are indicated above the lanes. Glycosylation results in a mobility shift from the non-glycosylated (g0) to the glycosylated form of the acceptor protein (g1). Functional PglB is partially auto-glycosylated at N535 and N556, resulting in two additional bands (g1 and g2). ( c ) Influence of different divalent metal cations on in vitro activity of PglB. The turnover rate of PglB devoid of the His 10 affinity tag on fluorescently labelled substrate peptide (DQ N AT sequon) was determined at various concentrations of different divalent metal cations. The activity profile at 0.1 mM metal concentration is magnified in the inlet. ( d ) pH activity profile of PglB. The turnover rate of PglB on fluorescently labelled substrate peptide (DQ N AT sequon) was determined at various pH values and the obtained data were fitted with a function describing a bell-shaped pH curve ( R 2 =0.976). The calculated pK a values are indicated. ( c , d ) Each data point results from a single turnover rate determination and the error bars account for the s.e.m. of each fit. Full size image Various acidic residues at the active site have been shown to be important for PglB function in vivo and in vitro [15] , [16] , [29] including Asp56 and Glu319 but also Asp154 and Asp156. We found that individual mutations of Asp56 and Glu319 to alanines abolished sequon binding ( Supplementary Fig. S8 ) [15] . Replacement by iso-electronic amides (D56N and E319Q) had a slightly less severe effect, but peptide binding was still too weak to determine K d values ( Table 2 , Supplementary Fig. S8 ). Residues Asp154 and Asp156 constitute a DXD motif that is also present in other enzymes of the GT-C superfamily [30] , [31] . The carboxyl group of Asp154 is not directly involved in acceptor substrate binding but is coordinating the divalent metal ion, whereas Asp156 is probably involved in stabilizing the hydrogen-bonding network in the catalytic site ( Fig. 4a ). The mutations D154A, D154N, D156A and D156N also showed impaired peptide binding, with K d values ~40–90-fold higher than those for wt sequon ( Table 2 , Supplementary Fig. S8 ). Table 2 Dissociation constants for PglB active site mutants. Full size table When we quantified in vitro glycosylation rates for the above mutants, we realized that the most disfavoured mutants showed fluctuations in turnover of up to 15-fold, resulting in poor reproducibility between distinct protein preparations ( Supplementary Table S1 ). We found that the mutation D56A had the most severe reduction in activity (11,000–150,000-fold), followed by D154A (3,500–30,000-fold), E319A (900–1,000-fold) and D156A (450–500-fold). With the exception of D56N, individual replacements of the carboxyl groups by iso-electronic carboxamides resulted in a more pronounced reduction in activity than mutations to alanines. These findings illustrate that the negative charges provided by individual carboxyl groups are essential for catalysis and that steric effects might explain the additional decrease in activity for mutants D154N, D156N and E319Q. Unexpectedly, elevated concentrations of Mn 2+ did not increase the turnover rates of active site mutants. For example, the optimum Mn 2+ concentrations for Glu319 and Asp156 mutants were lower than those of wt enzyme ( Supplementary Fig. S9 ). Different divalent metal cations can serve as cofactors We previously reported that at the optimum metal concentration (20–50 mM), Mn 2+ yielded a threefold higher glycosylation rate than Mg 2+ , and that at lower, physiologically more relevant concentrations, Mg 2+ and Mn 2+ showed similar activities [15] . We now investigated PglB activity in the presence of Co 2+ , Ni 2+ and Zn 2+ . To prevent artefacts, we removed the His 10 affinity tag from PglB before functional analysis. The tag-less PglB protein yielded slight differences in the activity profiles for the various metal cofactors ( Fig. 4c ). The highest activity was observed at 10 mM Mn 2+ . Co 2+ yielded higher, whereas Ni 2+ and Zn 2+ generally yielded lower activities than Mg 2+ . However, at 0.1 mM concentration, Co 2+ , Ni 2+ and Zn 2+ yielded higher activities than Mg 2+ ( Fig. 4c ), suggesting that in vivo , these transition metals are potential candidates for OST cofactors. pH activity profile of PglB We determined the pH profile of PglB-mediated glycosylation in vitro using 10 mM Mn 2+ as cofactor. We observed a bell-shaped activity profile with an optimum at pH 6.8. Fitting the determined turnover rates resulted in p K a values of 4.7 and 8.0 ( Fig. 4d ). As the discovery of protein N-glycosylation is an essential post-translational modification in the secretory pathway of eukaryotic cells, the reaction mechanism of OST, specifically the activation of the carboxamide group of the acceptor asparagine, has been in dispute. Two fundamentally distinct activation mechanisms are outlined in Fig. 5 . The first hypothesis involves a general acid/base-driven activation, which represents a modified proposal based on Bause’s [17] suggestion that a catalytic base abstracts a proton from the hydroxyl group of the +2 Ser/Thr, triggering the deprotonation of the acceptor Asn side chain when in contact with the deprotonated +2 hydroxyl group. In line with hypothesis 1, Imperiali et al . [14] as well as Marshall [32] independently proposed that a catalytic base abstracts an amide proton, whereas the hydroxyl group of the +2 Ser/Thr serves as a hydrogen donor to the amide carbonyl oxygen. All three proposals require a catalytic base near the active site of the enzyme and rely on conformations that position the hydroxyl moiety of the +2 Ser/Thr in hydrogen-bonding distance to the Asn side chain amide. Whereas the second requirement was clearly incompatible with the X-ray structure of PglB, enolization of the carboxamide group, facilitated by a catalytic base, remained a possibility. Hypothesis 2 (twisted amide, Fig. 5 ) emerged from the PglB structure, in particular the close interaction of the metal ion, the catalytically essential carboxyl groups of Asp56 and Glu319 and the carboxamide group of the acceptor Asn. 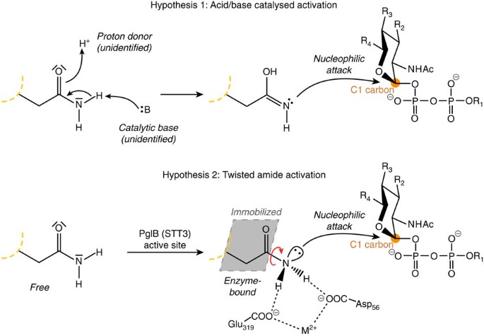Figure 5: Mechanistic hypotheses for catalytic activation of amide nitrogen. Yellow dashed lines indicate polypeptide backbone. Orange circles indicate the C1 carbon of the reducing end sugar. For hypothesis 1, protonation of the carbonyl oxygen and deprotonation of the amide nitrogen are indicated. For hypothesis 2, the acceptor Asn side chain is immobilized when bound to PglB (grey plane) and the amide group may form hydrogen bonds with residues D56 and E319, requiring rotation of the C-N bond (red arrow). R1: Dolichyl (eukaryotes), Undecaprenyl (bacteria); R2: OH (eukaryotes), Oligosaccharyl (bacteria); R3: Oligosaccharyl (eukaryotes), NHAc (bacteria); R4: CH2OH (eukaryotes), CH3(bacteria). Figure 5: Mechanistic hypotheses for catalytic activation of amide nitrogen. Yellow dashed lines indicate polypeptide backbone. Orange circles indicate the C1 carbon of the reducing end sugar. For hypothesis 1, protonation of the carbonyl oxygen and deprotonation of the amide nitrogen are indicated. For hypothesis 2, the acceptor Asn side chain is immobilized when bound to PglB (grey plane) and the amide group may form hydrogen bonds with residues D56 and E319, requiring rotation of the C-N bond (red arrow). R 1 : Dolichyl (eukaryotes), Undecaprenyl (bacteria); R 2 : OH (eukaryotes), Oligosaccharyl (bacteria); R 3 : Oligosaccharyl (eukaryotes), NHAc (bacteria); R 4 : CH 2 OH (eukaryotes), CH 3 (bacteria). Full size image We first ruled out an essential role of His485, the only residue close enough to the acceptor Asn that could serve as a proton acceptor in addition to Asp56 and Glu319, in PglB activity. Rather than a catalytic involvement, His485 appears to have a structural role in PglB. In principle, abstraction of a proton by residues Asp56 or Glu319 remained a possibility; however, this would require a rotation of the deprotonated carboxamide nitrogen to allow a nucleophilic attack on the LLO. We therefore characterized the roles of Asp56 and Glu319. Their carboxyl groups could in principle act as a catalytic base; however, because of their interactions with the bound divalent metal cation they probably only serve as hydrogen-bond acceptors ( Fig. 4a ). Individual mutations of Asp56 and Glu319 not only impaired catalysis but, more importantly, severely affected substrate peptide binding, suggesting that the carboxyl groups of both residues are indeed involved in amide binding even in the absence of LLO. The proposed hydrogen bonding illustrated in Fig. 5 is optimal when the C–N bond of the acceptor carboxamide group is rotated to generate a twisted amide. As depicted in Fig. 5 , such a distortion generates a reactive free electron pair at the nitrogen. Twisted amides are known to have a substantially higher reactivity than planar amides and were indeed proposed to have a role in biological reactions involving amide groups [33] , [34] , [35] . Backbone amide distortion has been described in crystal structures of proteins that undergo autoproteolysis [36] , [37] , and experimental data provide additional support that this unusual conformation of the scissile amide bond is the driving force for a nucleophilic attack during the catalysis of protein splicing [38] . These findings demonstrate that protein-catalysed reactions can indeed provide the energy required for amide C–N bond rotation, estimated to be ~16–20 kcal mol −1 (ref. 39 ). A twisted amide activation of Asn in PglB-catalysed N-glycosylation, facilitated by two strong hydrogen bonds provided by Asp56 and Glu319, can explain why the Dab-containing peptide analogue was an inhibitor in our in vitro assay and could not be glycosylated, even at elevated PglB concentrations, whereas the Hse-containing peptide was O-glycosylated. Unlike Hse, Dab is protonated at physiological pH and could only present a free electron pair following deprotonation. Given the free rotation around the C–N bond of the primary amine, Dab probably forms two hydrogen bonds, one each with Asp56 and Glu319. As a result, the electron density on the amine nitrogen of Dab will increase, making an abstraction of the remaining proton (and the generation of a reactive electron pair) impossible under conditions where PglB is active. It was somewhat unexpected that Dab had a lower binding affinity for PglB than the Asn-containing, wt sequon. There are two possible explanations. On one hand, the carbonyl group of the Asn side chain is likely interacting with PglB, although the detailed contacts are impossible to delineate at the present resolution of the structural information. On the other hand, the positive charge of the primary amine group could be weakening the binding to PglB. In comparison, the binding of the Hse substrate to PglB is probably weak because the hydroxyl group can only form one hydrogen bond (either with Asp56 or Glu319). However, Hse can provide relatively reactive electron pairs that can attack LLO, resulting in observable glycosylation. These findings support the notion that two hydrogen bond acceptors (Asp56 and Glu319) are essential for PglB activity and that no other base is required. We should emphasize that there are other factors that can increase the reactivity of the amide nitrogen—for example, the involvement of a nucleophile attacking the carbon atom of the C=O double bond. Similar to an addition reaction, this would effectively break the conjugation of the nitrogen electrons with the carbonyl group. At present, the resolution of the PglB structure is too low to identify potential water molecules that could serve this purpose. However, as indicated in Fig. 5 (hypothesis 2), it is essential that the carbonyl group is immobilized in the tunnel connecting the peptide-binding site and the catalytic pocket, although the details of the interactions require higher resolution to define. Replacing one of the amide protons by a methyl or an O-methyl substituent resulted in compounds 7 and 8, which could in principle be accommodated in the active site of PglB, provided the side-chain analogues are in the Z configuration. The fact that binding was abolished suggests that no hydrogen bonds were formed with Asp56 or Glu319. This may be because of steric constraints, which could also explain that not even traces of glycosylation were detected. By contrast, upon replacing an amide proton with a hydroxyl group (resulting in the hydroxamate Asp(NHOH, compound 6), we observed a sizeable binding affinity, suggesting that both the remaining proton and the hydroxyl group must form stabilizing interactions with PglB, in line with carboxamide twisting. For glycosylation, however, the hydroxamate does not need to be rotated, as the terminal hydroxyl group represents a highly reactive nucleophile because of the alpha effect [23] . This results in an unusual O-linked glycosylation reaction, as demonstrated by our NMR studies. Our experiments illustrated that of the 20 natural amino acids, only asparagine is able to bind efficiently to PglB. At the same time, we could rationalize glutamine N-glycosylation. The carboxamide group of Gln is expected to project ~1.5 Å beyond the optimal position in the active site of PglB because of the additional methylene group compared with Asn. As a result, a glutamine-containing acceptor sequon either positions the Gln–carboxamide group correctly for activation (and binding contributions), which disturbs the interactions between the acceptor peptide backbone and the PglB surface. Alternatively, if the acceptor peptide benefits from all binding interactions with PglB, the carboxamide group cannot be properly placed. This might explain why glycosylation of Gln was ~200,000-fold slower than that of Asn in vitro and why glycosylation of glutamines is very rare in vivo . Nevertheless, using advanced mass spectrometry techniques, ‘Q-linked’ glycosylation was demonstrated for the V L domain of an IgG2a antibody, which was glycosylated at Gln106 with an occupancy of 0.02% (ref. 40 ). The function of the divalent metal ion in PglB appears to be twofold. As is the case for soluble, metal-dependent glycosyltransferases, M 2+ is a Lewis acid stabilizing the lipid-pyrophosphate leaving group. In addition, it is a cofactor that stabilizes the conformation of functional residues and acceptor Asn in the catalytic site. Our finding that Mn 2+ and Mg 2+ can be replaced by other ions such as Co 2+ , Ni 2+ and Zn 2+ in vitro was unexpected. Even though the divalent cation radii for Co 2+ , Ni 2+ and Zn 2+ are between those of Mg 2+ (0.65 Å) and Mn 2+ (0.8 Å), and all five cations exhibit comparable coordination behaviour, a replacement of Mg 2+ or Mn 2+ by Zn 2+ is rather unusual for metal-dependent enzymes [41] , [42] , [43] . The importance of the metal ion might be reflected in the observed pH activity profile of PglB. The second p K a value of 8.0 probably reflects a reduced solubility of Mn 2+ at high pH—that is, the insolubility of Mn(OH) 2 . The determinant for the first p K a value of 4.7 is less clear. Besides the carboxyl groups of Asp56 and Glu319, Asp465 (which is part of the WWD motif) might be protonated. As Asp465 has a central role in binding +2 Ser/Thr of the acceptor sequons, it would lose its function as a hydrogen bond acceptor upon protonation [16] , [44] . The question arises why nature chose Asn over Gln for N-glycosylation. Whereas the frequencies of Asn and Gln in the proteomes of modern organisms are nearly identical, Asn was almost twice as abundant as Gln in ancient organisms, in which N-linked glycosylation probably originated [45] , [46] , [47] . The side chain of Asn also exhibits a smaller degree of flexibility than that of glutamine, providing entropic advantages for substrate binding and catalysis. Whatever the driving force for establishing the N-X-S/T sequon was, the same sequon was selected twice for the attachment of glycans in evolution [19] , [48] , [49] . It is possible that the biophysical properties of the N-X-S/T sequon are the basis of this convergent evolution. Alternatively, molecular mimicry might be the selective force leading to the generation of this N-glycosylation system in pathogenic bacteria. In the case of OST, a fascinating mechanism has evolved that accurately distinguishes Gln from Asn residues but uses the carboxamide group both for substrate binding and efficient catalytic activation. Along with the Asn side chain, the hydroxyl-containing amino acid (Ser/Thr) in the +2 position provides enough selectivity and binding energy for efficient selection and glycosylation of the entire substrate repertoire of a cell. In combination with the high stability of the N-glycosidic linkage, these features are the basis of the high abundance of N-glycoproteins in all domains of life. Reagents All reagents were purchased from Sigma-Aldrich, Fluka, Acros Organics or Alfa Aesar. 5-Carboxyfluorescein (5-CF) was purchased either from Novabiochem (Switzerland) or from OChem Incorporation (USA). The amino-acid building blocks and PyBOP were purchased from Advanced ChemTech (USA) or Novabiochem (Switzerland). Fmoc-protected TentaGel S RAM resin was purchased from Rapp Polymere (Germany). Construction of plasmids Mutations in the pglB gene of C. lari were generated by the QuickChange method either on a pBAD plasmid [16] for in vitro glycosylation studies or on a pMLBAD plasmid [50] for in vivo glycosylation assays. For in vitro glycosylation, the two endogenous glycosylation sites were removed (N535Q, N556Q) to prevent auto-glycosylation of PglB. The resulting construct was referred to as wt construct and all subsequent mutations were based on this construct. Introduction of a 3C proteolytic cleavage site between the pglB gene and the polyhistidine tag was performed by ligation of phosphorylated, double-stranded DNA of oligonucleotides 5′-AATTCGGCAGCGGCCTGGAAGTCCTGTTTCAGGGTCCGG-3′ and 5′-AATTCCGGACCCTGAAACAGGACTTCCAGGCCGCTGCCG-3′ into the wt pBAD plasmid digested with the enzyme EcoR I. All plasmids were validated using DNA sequencing. In vivo glycosylation assay To analyse the activity of C. lari PglB mutants in vivo , E. coli SCM6 cells were transformed with three separate plasmids carrying the C. jejuni pglB mut cluster containing an inactivated pglB gene (W458A and D459A) [51] , the glycosylation acceptor protein 3D5 containing a DQNAT acceptor site [52] and C. lari PglB, wild-type or mutants. A 5-ml pre-culture was inoculated from a single clone and grown overnight at 37 °C in LB medium. The main culture was inoculated to an optical density (A 600 ) of 0.05 in 15 ml LB medium and grown at 37 °C to A 600 of 0.5. The culture was induced by the addition of arabinose to 0.1% (w/v) and grown for 4 h at 24 °C. For extraction of periplasmic proteins, an equivalent of 1 ml culture volume with an A 600 of 3 was collected using centrifugation, resuspended in 150 μl extraction buffer, consisting of 30 mM Tris-HCl, pH 8.5; 20% (w/v) sucrose; 1 mM EDTA and 1 mg ml −1 lysozyme (Sigma) and incubated for 1 h at 4 °C. A final centrifugation step yielded periplasmic proteins in the supernatant. Expression and glycosylation of the acceptor protein 3D5 was monitored using SDS–PAGE of periplasmic cell extracts and visualized by mobility shift to increased size in an immunoblot using an anti-c-Myc antibody, or by the reactivity of the glycoprotein in an anti-glycan Immunoblot using hR6 antiserum. Immunodetection of PglB expression was performed from whole-cell extracts using an anti-HA antiserum (Santa Cruz Biotechnology). All experiments were performed at least in triplicate, and representative samples are shown. Expression and purification of PglB mutants PglB mutants were overexpressed in E. coli BL-21 (DE3) Gold cells in a 30-l fermenter or in 5-l baffled flasks using Terrific Broth medium supplemented with 1% (w/v) glycerol. Cells were grown to A 600 of 10.0 (fermenter) or 3.0 (flasks) at 37 °C and induced with 0.1% (w/v) arabinose for 2 or 4 h, respectively. Cells were collected using centrifugation and pellets were stored at −80 °C before membrane preparation. Cell pellets were resuspended in 25 mM Tris-HCl, pH8.0; 250 mM NaCl and disrupted in a M-110L microfluidizer (Microfluidics) at 15,000 psi external pressure. Membranes were pelleted using ultracentrifugation at 100,000 g for 0.5 h. All subsequent steps were carried out at 4 °C. PglB was solubilized in 25 mM Tris-HCl pH 8.0, 250 mM NaCl, 10% (v/v) glycerol and 1% (w/v) n-dodecyl-β-D-maltopyranoside (Anatrace) for 1 h. All purification buffers contained n-dodecyl-β-D-maltopyranoside. PglB was purified on a NiNTA superflow affinity column (Qiagen) and desalted into 10 mM MES pH 6.5, 100 mM NaCl, 0.5 mM EDTA and 3% (v/v) glycerol. Desalted protein was analysed using size exclusion chromatography (Superdex 200, GE healthcare) and, if needed, concentrated up to 20 mg ml −1 in a 100 kDa molecular weight cutoff Ultra-15 concentrator (Amicon, Millipore). The concentrated sample was re-analysed using gel filtration, and protein concentrations were determined with A 280 using diluted samples. For purification of PglB with a cleavable polyhistidine tag, the protein was desalted into 25 mM Tris-HCl pH 8.0, 250 mM NaCl and 10% (v/v) glycerol and incubated with 3C protease (prepared in-house) in a 2:1 ratio (PglB:3C) for 2 h at 4 °C. The sample was supplemented with 10 mM imidazole and reloaded on a Ni-NTA affinity column. The flow through was collected, supplemented with 0.5 mM EDTA and desalted into 10 mM Mes pH 6.5, 100 mM NaCl and 3% (v/v) glycerol. Synthesis of fluorescein-labelled acceptor peptides Peptide synthesis was initiated by loading of TentaGel S RAM resin (500 mg, loading: 0.24 mmol g −1 ) in a 10-ml polypropylene syringe fitted with a polypropylene frit, a teflon stopcock and a stopper. The resin was swollen in DCM (6 ml, 20 min). After removal of the DCM, the Fmoc-protecting group of the resin was removed by using a solution of 20% piperidine in NMP. Stirring of the reaction mixture at any given step was performed by attaching the closed syringes to a rotating axis. The completion of the reaction was checked using the TNBS test. Removal of the Fmoc-protecting group was performed by using a solution of 20% piperidine in NMP (6 ml, 2 × 10 min). After filtration, the resin was washed with NMP (2 × 6 ml), MeOH (2 × 6 ml) and DCM (2 × 6 ml). Coupling of amino acids was performed by using Fmoc-protected amino acids (3 eq), PyBOP (3 eq) and DIEA (6 eq) in NMP (6 ml). The resin was stirred for 2 h before it was washed with NMP, MeOH and DCM (2 × 6 ml each). Acetylation of the resin was performed after each amino-acid coupling using a solution of acetic anhydride:DCM (1:1). Coupling of 5-CF was performed by using 5-CF (2 eq), HOBt (5 eq) and DIC (5 eq) in NMP (6 ml). The resin was stirred overnight and protected from light using aluminium foil. The resin was washed with NMP, MeOH and DCM (2 × 6 ml each). A solution of 20% piperidine in NMP (6 ml, 6 × 5 min) was added to the resin to remove the excess of free 5-CF before the resin was finally washed with DCM (6 × 6 ml). After coupling of the fluorophore, the compounds were protected from light with aluminium foil at all time. Trifluoroacetic acid (TFA) cleavage was performed by adding a solution of TFA/TIS/H 2 O (94:5:1, v/v/v) to the resin for 1 h. The peptide was precipitated with tert -butylmethylether and dissolved in H 2 O/MeCN with 0.1% TFA mixture. Labelled acceptor peptides were purified by preparative RP-HPLC and obtained as yellow foamy solid after lyophilization. For Allyl/Alloc deprotection, the polypropylene syringe was equipped with a septum and dried under high vacuum for 1 h, before it was swollen in dry DCM for 10 min under argon. After removal of the solvent, Pd(PPh 3 ) 4 (0.15 eq) and phenylsilane (15 eq) were diluted in 4 ml of dry DCM and added to the resin under argon. The reaction was stirred under argon bubbling for 20 min before the reagents were removed by filtration, and the resin was washed with dry DCM. The procedure was repeated once. Finally, the resin was washed with a sodium diethylcarbamate solution (0.02 M in DMF) and then with dry DCM (8 ml, 2 × 10 min). Peptides were dissolved to 2–5 mM in dimethylsulphoxide and the concentration of peptides was determined from a dilution in 100 mM Tris-HCl pH 9.0 by A 495 with an extinction coefficient of 79,000 M −1 cm −1 . A detailed description for the synthesis of individual peptides and amino-acid building blocks can be found in Supplementary Methods . Fluorescence anisotropy measurements Desalt buffer (70 μl) supplemented with 1 μM peptide substrate and 10 mM MnCl 2 was titrated with concentrated PglB containing equal concentrations of peptide substrate and MnCl 2 . Anisotropy was measured with a Quantamaster QM-7/2003 spectrofluorometer (Photon Technology International) in a T-format at 4 °C. Each concentration was measured 20 times for 1 s at 494 nm excitation and 521 nm emission wavelengths. Anisotropy was calculated using equation [1]. Anisotropy was plotted against total protein concentration and data were fitted in Prism (GraphPad Software) using equation [2] for the 1:1 stoichiometry. Protein solution from the cuvette was re-analysed using size exclusion chromatography after each anisotropy measurement to prove stability of the protein over the course of the experiment. Extraction of LLOs LLOs were extracted from E. coli SCM6 cells carrying the C. jejuni pglB mut cluster [51] (containing an inactivated pglB gene) by a mixture of Chloroform:MeOH:H 2 O=10:20:3 (ref. 53 ). Generation and isolation of LLOs with truncated glycan structures will be published elsewhere. Extracts were dried in a rotavap and reconstituted in a buffer containing 10 mM Mes pH 6.5, 100 mM NaCl and 1% Triton X-100 (w/v). The concentration of reconstituted LLOs was determined by titrating various amounts of LLO against a constant amount of acceptor peptide in an in vitro glycosylation assay. In vitro glycosylation assay In a reaction containing 10 mM Mes pH 6.5, 100 mM NaCl, 10 mM MnCl 2 , 3% glycerol (v/v) and 1% Triton X100 (w/v), 10% LLO extract (v/v, corresponding to 35 μM) and various amounts of PglB (1 nM–25 μM) were mixed. The mixture was pre-incubated at 30 °C in a water bath for 5 min before the reaction was started by addition of 10 μM fluorescently labelled acceptor peptide. Reactions were incubated in a water bath at 30 °C. Samples were taken at different time points and reactions were stopped by the addition of 4 × SDS sample buffer. Samples were diluted 200-fold prior to analysis by Tricine SDS–PAGE [54] . Fluorescent bands for peptide and glycopeptide were visualized by using a Typhoon Trio Plus imager (GE Healthcare) with excitation at 488 nm and a 526-nm SP emission filter. The amount of formed glycopeptide was determined from band intensities of fluorescence gel scans (ImageJ), in which the sum of signals for glycosylated and non-glycosylated peptides for each lane was defined as 100%. For turnover rate determination, a total of five samples were taken in 6-min intervals and data were fitted using linear regression. For M 2+ titration experiments, PglB (4 nM wt enzyme and 0.5–25 μM mutant enzyme) was incubated with various amounts of CoCl 2 MgCl 2 , MnCl 2 , NiCl 2 and ZnCl 2 , respectively. Four samples were taken at appropriate time intervals (2–16 min) so that the reaction was in a linear range. Data were fitted using linear regression to determine turnover rates. For pH activity profile determination, 4 nM PglB wt enzyme was incubated in a reaction mix containing 20 mM of different buffers. The pH of each condition was determined (NaAc pH 4.2 and pH 4.9; Mes pH 5.5 and pH 6.1; Pipes pH 6.5; Hepes pH 7.3; Tris pH 8.2; Glycine pH 8.6; Caps pH 8.8), and four samples were taken at appropriate time intervals (2–20 min) so that the reaction was in a linear range. Data were fitted using linear regression to determine turnover rates. Obtained rates were plotted against pH values and data were fitted in Prism (GraphPad Software) using equation [3]. Endoglycosidase treatment and extraction of glycopeptides For endoglycosidase treatment, a reaction containing 1 nmol glycopeptide was supplemented with 15 μg bovine serum albumin and incubated with 100 U α- N -Acetyl-galactosamininidase for 4 h at 37 °C. Extraction of glycopeptides from the in vitro glycosylation reaction was performed by the addition of 1 ml of 3:2 chloroform:methanol and 200 ml of 4 mM MgCl 2 as described before [55] , and extracted peptides were dried in a speed vac. For fluorescence anisotropy measurements, samples were dissolved in ddH 2 O and the concentration of glycopeptides was determined with the absorbance at 495 nm (see above). For NMR analysis, the extracted glycopeptide was extensively dialysed against ddH 2 O using a Cellu·Sep membrane (1.0 kDa MWCO, Membrane Filtration Products, Inc.) before it was lyophilized and dissolved in D 2 O. Mass spectrometry Fluorescently labelled substrate peptides containing either a DQNAT or a DQQAT sequon were extracted from in vitro glycosylation reactions and subjected to nanoLC-ESI-MS/MS analysis. Samples were desalted using C18 Zip-tip and loaded on an Eksigent nano-HPLC system using an auto sampler with a self-made reverse-phase tip column (75 μm × 80 mm) packed with C18 material (AQ, 3 μm, 200 Å; Bischoff GmbH). The gradient consisted of 10–30% acetonitrile (ACN) in 0.2% formic acid (FA) at a flow rate of 250 nl min −1 for 60 min and 30–50% ACN in 0.2% FA for 5 min. High accuracy mass spectra were acquired with an LTQ Orbitrap Velos mass spectrometer (Thermo Fisher Scientific) in the mass range of m/z 300–2,000 at a resolution of 60,000 at m/z 400 and a target value of 1 × 10 6 ions. Inclusion parent list was used to set normalized collision energy 35% for glycopeptides at MS1 mass of m/z 872.9149 and normalized collision energy 55% at MS2 mass of m/z 1,439.2780. Minimum signal required for triggering MS3 was set at a threshold of 1 × 10 3 ions. Peptides containing Asp(NHOH) (compound 6) were extracted from the in vitro glycosylation reaction, desalted with a C18 ZipTip and eluted with 70% ACN and 0.1% FA. Peptides were mixed at a ratio of 1:1 with α-cyano-4-hydroxycinnamic acid (5 mg ml −1 in 70% ACN and 0.1% TFA) as a matrix for spotting on the target plate. Peptides were analysed on MALDI-TOF/TOF 4800 proteomics analyser (Applied Biosystems) operated in the positive reflectron mode. NMR spectroscopy All spectra were recorded on a Bruker Avance III 500 or 900 MHz spectrometer at 293 K unless stated otherwise. The peptide containing unmodified Asp(NHOH) (compound 6) was dissolved in D 2 O at a concentration of 0.5 mM. The reaction product of the in vitro glycosylation of compound 6 was extracted, dialysed, lyophilized and dissolved in 250 μl D 2 O at a concentration of 0.35 mM. A 2D NOESY spectrum was recorded at 900 MHz with a mixing time of 150 ms, 96 transients and 2,048 × 674 points. 2D TOCSY spectra were recorded at 900 MHz with mixing times of either 13 or 80 ms, 4 transients and 2,048 × 512 points. 1 H– 13 C HSQC spectra were recorded at 283 K with typically 260 transients and 2,048 × 220 points. Spectra were processed using Topspin 2.1 (Bruker) and analysed with Sparky (Goddard, T.D. & Kneller, D.G. SPARKY 3. University of California, San Francisco). All spectra were referenced to DSS according to Markley et al . [56] Assigning the C1 chemical shift of diNAcBac In an 1 H– 13 C HSQC spectrum of the in vitro glycosylated Asp(NHOH) peptide (natural abundance 13 C), almost all correlations of the C. jejuni N-glycan are observed except the characteristic C1–H1 correlation of diNAcBac linked to Asn at 80.8 p.p.m. (ref. 18 ). To unambiguously assign the H1 of diNAcBac, we first recorded a 2D NOESY spectrum ( Supplementary Fig. S4 ). The isolated chemical shift of the diNAcBac methyl group of C6 at ~1.1 p.p.m. shows normally two strong NOE cross-peaks within the anomeric region: an inter-residual NOE to GalNAc2 H1 and an intra-residual NOE to diNAcBac H1 (ref. 18 ). Most NOE cross-peaks of in vitro glycosylated Asp(NHOH) peptide and the in vitro glycosylated protein AcrA61-210ΔΔ are identical. However, H1 of diNAcBac resonates at 4.75 p.p.m. instead of 5.03 p.p.m. (ref. 18 ). The H1 resonance assignment of diNAcBac in the glycosylated Asp(NHOH) peptide was confirmed with 2D TOCSY spectra with different mixing times that display cross-peaks to other resonances of the spin system. In the initial 1 H– 13 C HSQC spectrum recorded at 293 K, artefacts around the residual HDO signal at 4.83 p.p.m. hampered the observation of a C1–H1 correlation and therefore another 1 H– 13 C HSQC spectrum was measured at 283 K (HDO at 4.95 p.p.m.). 2D TOCSY spectra recorded at 283 K revealed that the resonance of H1 did not change compared with spectra at 293 K. Only one C1–H1 correlation is found at the H1 resonance of diNAcBac so that C1 can be assigned to 106.4 p.p.m. This value fits well to previously reported chemical shifts of glycosyl hydroxamates. For example, a lactose hydroxamate shows a C1 chemical shift of 106.0 p.p.m. (referenced to TSP that is comparable to DSS) [21] and glucose hydroxamate of Trichostatin C displaying a C1 resonance at 107.9 p.p.m. (referenced to TMS, corresponding to 106.3 p.p.m. against DSS) [22] . How to cite this article: Lizak, C. et al . Unexpected reactivity and mechanism of carboxamide activation in bacterial N-linked protein glycosylation. Nat. Commun. 4:2627 doi: 10.1038/ncomms3627 (2013).